Approaching the ideal elastic limit of metallic glasses The ideal elastic limit is the upper bound to the stress and elastic strain a material can withstand. This intrinsic property has been widely studied for crystalline metals, both theoretically and experimentally. For metallic glasses, however, the ideal elastic limit remains poorly characterized and understood. Here we show that the elastic strain limit and the corresponding strength of submicron-sized metallic glass specimens are about twice as high as the already impressive elastic limit observed in bulk metallic glass samples, in line with model predictions of the ideal elastic limit of metallic glasses. We achieve this by employing an in situ transmission electron microscope tensile deformation technique. Furthermore, we propose an alternative mechanism for the apparent 'work hardening' behaviour observed in the tensile stress–strain curves. The familiar metals and alloys in our daily lives are all crystalline materials. In recent years, amorphous alloys, or metallic glasses (MGs), have emerged as a new category of advanced materials. A striking property of MGs is their high elastic limit far above that of their crystalline counterparts [1] , [2] , [3] . At room temperature, most MGs exhibit uniaxial yield stress ( σ y ) on the gigapascal level, and the corresponding yield strain ( ɛ y ) is as large as, almost universally, ~2% [2] . In comparison with common engineering materials [3] , the superior σ y and ɛ y of MGs clearly stand out (see comparison in ref. 3 ). Yet, these apparent values for σ y and ɛ y , though high, are actually not the ceiling, or ideal limit, for MGs. The observed onset of yielding in bulk MGs [2] is known to be controlled by the relatively easy propagation of shear bands [4] , [5] , which is the dominant mode of plastic deformation at temperatures well below the glass transition temperature ( T g ). Shear bands readily nucleate from preferential sites inevitably present in the as-prepared bulk MGs (including casting pores/flaws, surface notches and other stress concentrators). Barring such 'heterogeneous nucleation' assisted by extrinsic factors, the σ y and ɛ y ought to be higher. Moreover, in the amorphous structure there are internal 'defects' or inherently more fertile sites for shear transformations, and their coordinated organization/evolution can lead to the formation of shear bands [4] , [5] , [6] . This is analogous to the case of crystalline metals: normally there are pre-existing dislocations and easy sources for dislocation nucleation; in their absence yielding can be delayed so much that the elastic limit can be pushed towards the 'theoretical strength', which is at least an order of magnitude higher than the commonly observed apparent σ y . For example, it is well known that small volume single crystalline samples, such as whiskers [7] , nanowires [8] and nanopillars [9] , offer the opportunity to observe ultrahigh strength and large elastic strains close to the theoretical limit [10] . This is because only for such micro- and nano-scale samples can pristine crystals be made to minimize those defects that are inevitable in their bulk counterpart, such that nucleation of fresh defects is often required for yielding. The same strategy can be applied to MGs, by using micro- and nano-scale samples. In such samples the extrinsic flaws that concentrate stresses and facilitate shear banding are eliminated. In addition, internal structural defects become low in population and small in size, and are thus less probable to launch cooperative actions. As a result, shear banding [4] , [5] tends to be delayed. This should allow us to answer the question as to what the ideal strength (and elastic strain limit) is for MGs, and observe how close to it one can reach in experiments. This ultimate ceiling is of obvious interest for applications requiring high load-bearing capability and involving storage of elastic energy. Gaining quantitative and dynamical knowledge of the elastic behaviour on the submicron scale is, from a physics perspective, of paramount importance. In fact, information on elasticity at that length scale is perhaps more important than plasticity, as they are a direct reflection of the inherent structure of the glass. In this work, we choose to dynamically examine MG samples with the effective sample size, d , in the 200–300 nm regime, to uncover the ideal elastic limit at room temperature. This d range was chosen because, at larger sizes (for example, d >500 nm), the apparent strength would depend on d : σ y increases significantly with decreasing sample size and the ceiling has not been reached yet, as revealed by the tensile test inside a scanning electron microscope (SEM) [11] . When the sample sizes are extremely small (for example, d <100 nm), there can be major influences from surface conditions and surface diffusion, together with changes in the mode of plastic flow to include large elongation and necking [11] , [12] . This would make it difficult to compare with bulk samples and to determine sample cross-sectional area via postmortem SEM measurements. Previous experiments on submicron MG samples [6] , [11] , [12] , [13] , [14] , [15] , [16] , [17] , [18] , [19] , [20] , [21] have focused on the mode of plastic deformation and the plastic strain achievable, not dynamic elastic strain measurements and elastic limit. In addition, the in situ transmission electron microscopy (TEM) tensile tests using 'window-frame' rather than free-standing samples, are complicated by confinements/constraints and the lack of quantitative stress–strain curves [13] , [22] . 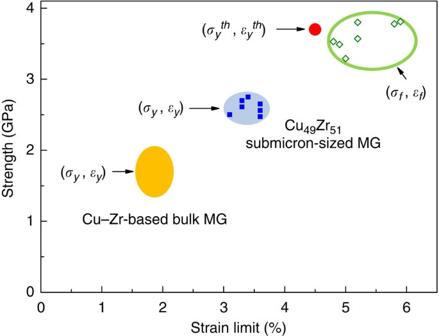Figure 1: Strength and strain limit of Cu–Zr metallic glasses. The yellow shaded ellipse area represents the yield stress and yield strain range of Cu–Zr-based bulk samples. All other data are results from ourin situtensile tests of Cu49Zr51samples with diameters in the range of 200–300 nm. The blue solid squares represent the yield strength (σy) and yield strain (ɛy) at the proportionality limit. The measured fracture strength (σf) and fracture strain (ɛf) are shown with green open diamonds. The theoretical elastic limit (σyth, ɛyth) given by equation (1) is marked by the red solid circle. Theɛfvalues exceed the theoretical elastic limit due to a small contribution from plastic deformation. When the latter (<1%) is deducted fromɛf, the resulting total elastic strain is consistent with the predicted ideal elastic strain limit. In situ tensile tests For comparison with the known properties of bulk MG samples, we first present in Figure 1 the typical range of σ y and ɛ y observed so far in compression tests of MGs, particularly those based on Cu–Zr alloys (yellow shaded region) [2] , [23] , [24] , [25] , [26] . This sets the stage for presenting the extraordinarily high-elastic limits discovered in the following from the submicron-sized MG samples. Figure 1: Strength and strain limit of Cu–Zr metallic glasses. The yellow shaded ellipse area represents the yield stress and yield strain range of Cu–Zr-based bulk samples. All other data are results from our in situ tensile tests of Cu 49 Zr 51 samples with diameters in the range of 200–300 nm. The blue solid squares represent the yield strength ( σ y ) and yield strain ( ɛ y ) at the proportionality limit. The measured fracture strength ( σ f ) and fracture strain ( ɛ f ) are shown with green open diamonds. The theoretical elastic limit (σ y th , ɛ y th ) given by equation (1) is marked by the red solid circle. The ɛ f values exceed the theoretical elastic limit due to a small contribution from plastic deformation. When the latter (<1%) is deducted from ɛ f , the resulting total elastic strain is consistent with the predicted ideal elastic strain limit. Full size image The material used for testing is a Cu 49 Zr 51 MG, prepared using melt spinning. 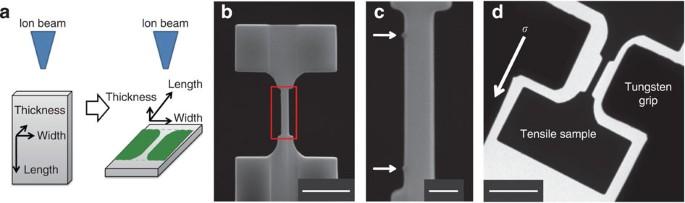Figure 2: Tensile specimen preparation and experimental setup. (a) Schematic representation of the FIB procedure for cutting the tensile samples. First a thin plate with dimensions of 400 nm (thickness)×2.5 μm (width)×5 μm (length) was FIB milled from its bulk parent body, with ion beam going through the length direction (left panel). Then a tensile sample was milled into the plate and the ion beam was parallel to the thickness direction (right panel). (b) SEM image of a typical as-fabricated tensile sample. The part framed by the red rectangular box is enlarged inc. The two markers that are critical for the following strain measurement were made by e-beam-induced carbon deposition, as indicated by the white arrows. (d) Low-magnification TEM image showing the experimental setup including the sample, the tungsten grip and the loading direction. The scale bars inb,canddrepresent 1 μm, 200 nm and 1 μm, respectively. Figure 2a is a schematic showing how a tensile specimen was prepared using focused ion beam (FIB) micromachining. The sample was FIBed from the MG parent body, and the T-shaped free end (upper part in Fig. 2b ) will be grabbed by the tungsten grip for tensile test. Figure 2c shows the two very small markers (indicated by white arrows) that define the gauge length. These markers were made by electron beam-induced carbon deposition in the FIB chamber. As detailed later, these fiduciary markers are critical for reliably measuring the strain actually experienced by the gauge length. A TEM image showing the overall tensile test assembly is displayed in Figure 2d . Figure 2: Tensile specimen preparation and experimental setup. ( a ) Schematic representation of the FIB procedure for cutting the tensile samples. First a thin plate with dimensions of 400 nm (thickness)×2.5 μm (width)×5 μm (length) was FIB milled from its bulk parent body, with ion beam going through the length direction (left panel). Then a tensile sample was milled into the plate and the ion beam was parallel to the thickness direction (right panel). ( b ) SEM image of a typical as-fabricated tensile sample. The part framed by the red rectangular box is enlarged in c . The two markers that are critical for the following strain measurement were made by e-beam-induced carbon deposition, as indicated by the white arrows. ( d ) Low-magnification TEM image showing the experimental setup including the sample, the tungsten grip and the loading direction. The scale bars in b , c and d represent 1 μm, 200 nm and 1 μm, respectively. Full size image A total of seven specimens were tested using the Hysitron PI95 TEM PicoIndenter, see the Methods section for details. The sample evolution during the tests was recorded in movies (see an example in Supplementary Movie 1 ). 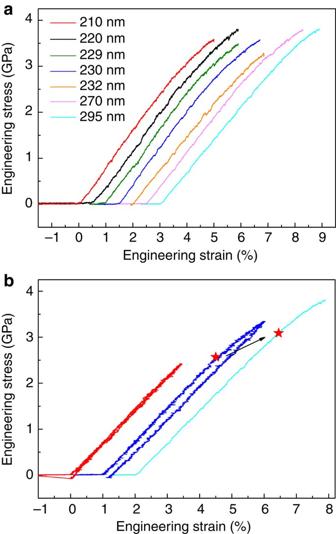Figure 3: Stress–strain curves from thein situtensile tests. (a) Engineering stress–strain curves of the seven specimens with different size and marked with different colours. They have been shifted relative to each other for the sake of clarity. (b) Three consecutive loading-unloading cycles were applied to thed=295 nm sample with a strain rate of about 2.3×10−3s−1. The first loading-unloading curve (red) exhibited completely linear elastic behaviour. Deviation from linearity was observed in the second loading cycle (dark blue) after the engineering strain reached ~3.6% (marked by a red star); ~5% total strain was applied in the second loading cycle and the unloading curve was quite linear. Approximately 0.3% residual plastic strain was observed at the end of this loading cycle. The sample fractured in the third loading cycle (light blue) when the strain reached ~5.9%. The yield stress indicated by the red star in the third loading cycle is higher than that in the second loading cycle. For comparison, the curves for the second and third loading cycles have been shifted. The resulting engineering stress–strain curves are shown in Figure 3a . These curves show good linearity in the early stage of loading, which is confirmed via multiple loading, unloading and reloading cycles, such as those displayed in Figure 3b . Interestingly, this apparent elastic region goes well beyond the yield point known for bulk-sized samples (including ribbons obtained by melt spinning) of this MG and similar MGs (the strength measured for bulk samples of this MG is in the range of 1.3–1.6 GPa, and elastic strain 1.7–2% [2] , [23] , [24] , [25] , [26] ). 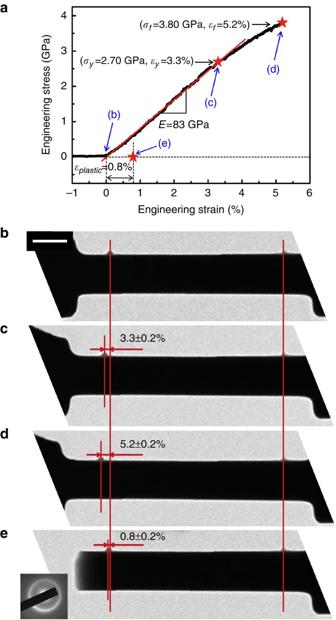Figure 4: Tensile behaviour and corresponding strain evolution of thed=220 nm sample. (a) Engineering stress–strain curve from the tension test. The average strain rate was about 2×10−3s−1. Mechanical properties extracted from the stress–strain curve include Young's modulus (E),σyandɛy(defined at the proportionality limit), fracture strength (σf) and total elongation to failure (ɛf), as well as the plastic strain (ɛplastic) remained in the gauge length. (b–e) These still frames extracted from the recorded movie (see corresponding points ina) demonstrate that the virgin sample (b) was elongated to a strain ofɛy=3.3±0.2% (c) when global yield began, and then fractured upon a total strain ofɛf=5.2±0.2% (d), among whichɛplastic=0.8±0.2% was measured frome, and the rest 4.4±0.2% was the total recoverable elastic strain. These strains were determined with high accuracy because there were no rough/irregular fracture surfaces to re-connect back, as the fracture occurred outside the section between the two markers. No crystallization was observed near the fractured region, as further confirmed by the selected area electron diffraction pattern (inset ofe) taken from the fractured area. The scale bar inbrepresents 200 nm, and the magnification was same for all the TEM images. Figure 4a illustrates the properties that were extracted from the curve, including the Young's modulus ( E ), σ y and ɛ y (defined here using the proportionality limit), as well as the fracture strength ( σ f ) and total elongation to failure ( ɛ f ). The E =83 GPa is similar to the values reported before for bulk samples of this MG (mostly in the 78 to 87 GPa range) [23] , [24] , [25] , [26] , whereas all the other properties are significantly higher. These results are not sensitively dependent on d in the d =200–300 nm regime. Figure 3: Stress–strain curves from the in situ tensile tests. ( a ) Engineering stress–strain curves of the seven specimens with different size and marked with different colours. They have been shifted relative to each other for the sake of clarity. ( b ) Three consecutive loading-unloading cycles were applied to the d =295 nm sample with a strain rate of about 2.3×10 −3 s −1 . The first loading-unloading curve (red) exhibited completely linear elastic behaviour. Deviation from linearity was observed in the second loading cycle (dark blue) after the engineering strain reached ~3.6% (marked by a red star); ~5% total strain was applied in the second loading cycle and the unloading curve was quite linear. Approximately 0.3% residual plastic strain was observed at the end of this loading cycle. The sample fractured in the third loading cycle (light blue) when the strain reached ~5.9%. The yield stress indicated by the red star in the third loading cycle is higher than that in the second loading cycle. For comparison, the curves for the second and third loading cycles have been shifted. Full size image Figure 4: Tensile behaviour and corresponding strain evolution of the d =220 nm sample. ( a ) Engineering stress–strain curve from the tension test. The average strain rate was about 2×10 −3 s −1 . Mechanical properties extracted from the stress–strain curve include Young's modulus ( E ), σ y and ɛ y (defined at the proportionality limit), fracture strength ( σ f ) and total elongation to failure ( ɛ f ), as well as the plastic strain ( ɛ plastic ) remained in the gauge length. ( b – e ) These still frames extracted from the recorded movie (see corresponding points in a ) demonstrate that the virgin sample ( b ) was elongated to a strain of ɛ y =3.3±0.2% ( c ) when global yield began, and then fractured upon a total strain of ɛ f =5.2±0.2% ( d ), among which ɛ plastic =0.8±0.2% was measured from e , and the rest 4.4±0.2% was the total recoverable elastic strain. These strains were determined with high accuracy because there were no rough/irregular fracture surfaces to re-connect back, as the fracture occurred outside the section between the two markers. No crystallization was observed near the fractured region, as further confirmed by the selected area electron diffraction pattern (inset of e ) taken from the fractured area. The scale bar in b represents 200 nm, and the magnification was same for all the TEM images. Full size image Additional elastic strain beyond proportionality limit Also, as indicated in Figure 4a , there appears to be an additional elastic strain that was sustained in the sample, after the onset of yielding. This was measured as follows: after fracture ( ɛ f =5.2%), the sample gauge length was found to have retained 0.8% plastic strain, as detailed in Figure 4b-e using the still frames extracted from the acquired TEM movie (see Supplementary Movie 1 ). Therefore 4.4% of the total strain was recovered upon unloading, significantly higher than the ɛ y =3.3% shown in Figure 4a . In other words, after the stress–strain curve deviates away from linearity, part of the ensuing deformation is from additional elastic deformation. This extra elastic strain is 4.4–3.3%=1.1%, and the (accompanying) plastic deformation is 5.2–4.4%=0.8%. The observation that the unloading curve shown in Figure 3b (second loading cycle, dark blue colour) is quite linear suggested that nonlinear elastic strain may not have a major role in the total strain. No obvious crystallization was observed in the regions near the fractured surface; see the selected area diffraction pattern (inset in Fig. 4e ). Comparison with bulk values The measured strain limits, σ y and ɛ y , as well as the σ f and ɛ f , have been added into Figure 1 . On average, these data points indicate an impressive ɛ y of 3.5±0.3%, and ɛ f of 5.3±0.4% (this latter value contains a small plastic strain, for example, a fraction of ~1%, as discussed above). The strengths achieved for this material are unprecedented as well, except for confined conditions under nanoindenter [27] , [28] . For example, σ y is ~2.7 GPa, and σ f is of the order of 3.8 GPa ( Fig. 4a ). These properties are about twice as high as those observed for bulk samples of this MG (yellow region in Fig. 1 ). Comparison with theoretical elastic limit We next compare the measured properties with the theoretical elastic limit estimated from modelling. For bulk MG samples, Johnson and Samwer [2] proposed an equation to describe the temperature-dependent shear strain limit, γ Y = γ C 0 − γ C 1 ( T / T g ) m , where γ Y is the elastic strain limit in shear, m is a scaling constant (2/3 in their model). Our comparison will be made at a typically used strain rate of ~10 −3 s −1 and T < T g . In such a regime γ C 0 =0.036 and γ C 1 =0.016 are constants obtained by fitting experimental data of elastic limit [2] , which, as discussed earlier, were determined by shear band propagation in bulk samples (the blue curve in Fig. 5 represents this scenario). The same equation has recently been confirmed [29] by analysis of atomistic calculations to be applicable for ideal elastic limit for yielding, but the fitting parameters were found to change to γ C 0 =0.11 and γ C 1 =0.09 (ref. 29 ). As MGs are isotropic and the Poisson's ratio for our MG is ν =0.36 (ref. 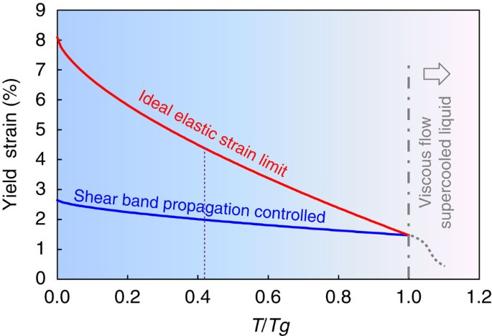Figure 5: The predicted elastic strain limit of Cu–Zr MG as a function of temperature. The strain rate is assumed to be 10−3s−1under uniaxial loading. The purple dashed line marks room temperature at which our experiments were carried out. The blue curve is for the elastic strain measured at yielding for bulk samples, where shear bands nucleate heterogeneously and the elastic limit is controlled by shear band propagation (for example, ~2% at room temperature), whereas the red curve is the prediction given by Equation (1) (for example, ~4.5% at room temperature), when shear band has to nucleate 'homogeneously' with little or no help from preferential sites29. The ceiling (red curve) can be achieved or approached in submicron-sized samples. The space between the two curves is the yield strain that can be possibly reached in experiments. 23 ), the above equation can be converted to obtain ideal strain limit in uniaxial loading using ɛ y = γ Y /(1+ν): This prediction of ideal elastic limit is shown using the red curve in Figure 5 for the Cu–Zr MG. At room temperature ( T =300 K), and taking T g =~730 K [23] , the ideal ɛ y of this MG is predicted to be 4.5%, and this corresponds to a σ y of 3.7 GPa for E =83 GPa. This point is also marked in Figure 1 (red solid circle). Figure 5: The predicted elastic strain limit of Cu–Zr MG as a function of temperature. The strain rate is assumed to be 10 −3 s −1 under uniaxial loading. The purple dashed line marks room temperature at which our experiments were carried out. The blue curve is for the elastic strain measured at yielding for bulk samples, where shear bands nucleate heterogeneously and the elastic limit is controlled by shear band propagation (for example, ~2% at room temperature), whereas the red curve is the prediction given by Equation (1) (for example, ~4.5% at room temperature), when shear band has to nucleate 'homogeneously' with little or no help from preferential sites [29] . The ceiling (red curve) can be achieved or approached in submicron-sized samples. The space between the two curves is the yield strain that can be possibly reached in experiments. Full size image Compared with the ~2% measured in bulk samples (see the room-temperature value on the blue curve in Fig. 5 ), the proportionality limit of ~3.5% observed in our 200–300 nm samples is closer to the ideal elastic limit of the MG. In addition, the ɛ f of ~5.3%, when the small (less than 1%, Fig. 4 ) accompanying plastic strain is deducted from it, in fact gives a total elastic (reversible) strain that is very close to the theoretical prediction from equation (1), that is, 4.5% (see the room-temperature value on the red curve in Fig. 5 ). The small plastic strain involved between ɛ y and ɛ f is very likely related to the fact that our free-standing samples all have surfaces. A surface is an imperfection in itself that may eventually become the preferred site for the initiation of plastic flow, such that the theoretical ɛ y of 4.5% may not be reached. In a molecular dynamics simulation, it was found that a MG with free surfaces yields at a strength ~15% lower than the same MG under periodic boundary conditions [29] . We note that the flow stress rises continuously with continued straining, as shown in Figure 3 . Such behaviour was not observed in bulk samples and could be perceived as the material undergoing fast 'work hardening' [11] . A likely origin of this behaviour, we speculate, is the delayed shear band nucleation, due to the small sample size. Specifically, in a free-standing sample without pre-existing flaws, the measured ɛ y (corresponding to the onset of plastic flow catalysed by the surfaces) would approach, but not reach, the ideal elastic limit. Different from a crystal, where dislocation nucleation is a highly localized event, a well-defined shear band from the surface in a free-standing MG may require a certain length scale to develop. As discussed by Shimizu et al . [4] , [5] and Shan et al ., [6] such a length scale is of the order of 10 2 nm, below which the groups of shear transformation zones (STZs) do not achieve the large aspect ratio needed for sufficient stress concentration to launch shear bands beyond their embryonic stages. As a result, our samples (200 nm~300 nm) may not undergo shear banding immediately after the onset of STZ activities from some local regions (for example, softer regions at or near surfaces). The sample is still dominated by harder and confined regions that continue to deform elastically, long after some STZs have started changing their configurations in a small fraction of the sample volume to bend the stress–strain curve (contributing small plastic strains, of the order of a fraction of 1% before fracture, see discussions earlier). One typical example is shown in Figure 3b . Most of the preferential STZ sites used up are not recovered after unloading (for example, Fig. 3b , second loading cycle). Upon reloading, higher yield stress is required to activate harder sites gradually to carry plastic relaxation through shear transformations (for example, Fig. 3b , third loading segment). The bending of the curve involving harder and harder regions can thus been envisioned as a manifestation of the inherently non-equilibrium and non-uniform (different degrees of local order) glassy structure. The increasing stress (from σ y to σ f ) sustains this coexisting elastic and plastic deformation, thereby exhibiting a regime of apparent 'work hardening'. Although the easy sites are being exhausted, the stress eventually becomes sufficiently high to drive STZ transformations all over the sample such that the latter as a whole enters the state of plastic flow. At that point, the lack of inherent microstructural work-hardening capability in an already plastically deformed glass triggers instability, which sets in by the formation of a major shear band (at σ f ), leading quickly to fracture to terminate the stress–strain curve. This line of reasoning, while only describing one possible 'work hardening' scenario, can rationalize why the yield stress increases with the additional loading cycles for the same sample ( Fig. 3b ) and why the apparent flow stress increases significantly with strain. Thus, our experiments effectively characterize the spectral width of the distribution of intrinsic strengths of STZs in a disordered metal. We note that MGs, which are inherently heterogeneous containing softer and harder local regions as mentioned earlier, are fundamentally viscoelastic [30] . However, they behave effectively elastic, as addressed in this paper, for deformation at room temperature (well below Tg) and normal strain rates 2 . In summary, our in situ and quantitative measurements using small MG samples reveal much-elevated elastic strain limits and corresponding stresses, compared with bulk samples. Before reaching σ f the total recoverable elastic strain (for example, Fig. 4 ) is consistently higher than the observed ɛ y at the proportionality limit. This maximum elastic strain achievable in the sample (for example, ~4.4% in Fig. 4 ), obtained after correcting ɛ f for the small plastic strain (<1%) it contains, is indeed very close to the predicted theoretical limit (the ideal ceiling of ~4.5% predicted by equation (1), see Fig. 5 ). The high elastic limit discovered in submicron samples is attractive for enhancing the applications of MGs, for example in microelectromechanical systems and nanoelectromechanical systems. Sample preparation The following procedure has been adopted to prepare the tensile samples: first a thin plate with dimensions of 400 nm (thickness)×2. 5 μm (width)×5 μm (length) was FIBed from its bulk parent body. Then a tensile sample was milled into the plate, and the sample gauge was trimmed to approach the designed width and length. Finally, the sample (mainly the gauge part) was further polished to reach the desired thickness with the ion beam at 30 kV / 5 pA as the final cutting condition. To keep the cross-section of the sample gauge uniform in thickness direction, the stage was tilted by one degree to compensate for the conical-shape ion beam profile upon the thinning of both sides of the sample. An SEM view of a typical specimen is shown in Figure 2b . Two markers, which are critical for accurate strain measurements, were made by e-beam-induced carbon deposition. This carbon deposition is usually deemed unwanted contamination, but is exploited here to provide well-defined fiduciary markers, as indicated by the white arrows in Figure 2c . Data acquisition and analysis In our work, the uniaxial tensile testing of individual stand-alone samples was accomplished quantitatively inside a TEM, taking advantage of the accurate displacement and load measurement capabilities of the Hysitron PI95 TEM PicoIndenter [31] , [32] . The real-time movies (for example, Supplementary Movie 1 ) of the tensile elongation of the sample were captured in situ in a JEOL-2100 field emission gun TEM operating at 200 kV. Occasional jerky shifts in the movie are not the real jerky slip of the tested sample, but image shift due to occasional discharging inside our instrument, as was supported by the following observations. First, there is no relative position change between the specimen and the grip during the image flash (and back). Second, the recorded load-displacement curves are quite smooth upon the jerky shifts. The average strain rate was about 2×10 −3 s −1 . Of the seven samples in Figure 3a , two of them (210 nm and 220 nm) have markers and three (232 nm, 270 nm and 295 nm) do not. To identify the e-beam effect on the testing results, the other two (229 nm and 230 nm) were tested with the e-beam blocked off. For all the samples, stress is calculated through dividing load by cross-sectional area. The cross-sectional area ( A ) of each specimen was measured from SEM images of the postmortem samples, see Supplementary Figure S1 . Such a measurement is reliable because the strain incurred in the sample is small and predominantly elastic. Therefore the A should be close to constant during and after the tensile test. The effective sample size diameter, d , is taken to be For samples with markers that define the gauge length, strains were accurately determined by measuring the changes between the deposited carbon markers (see Fig. 2c and Fig. 4b-e ), from the still frames extracted from the corresponding movies. For samples without markers, the uniform middle section of the sample is taken as the gauge length. Its change in the recorded movie was used to measure the strain. As the two ends in such gauges were not as well defined as in the marker cases, the strains determined would not be as accurate. For the determination of Young's modulus, we rely on the stress–strain curves (that is measuring the slope of their linear elastic portion) achieved from the samples with markers. Electron beam effect It should be noted that our experiments ruled out electron beam effects on the measured properties. For the comparative experiment on electron beam effect, three samples (see Supplementary Fig. S2 ) with identical projected geometry (along electron beam direction) were selected. Therefore, the gauge length of these three samples should be identical. The variation in diameter is due to the thickness difference. Consequently, if there is any obvious beam effect, the stress versus displacement curves of these three samples should be different. However, as one sees clearly from Supplementary Fig. S2 , the two samples tested with beam off displayed curves very similar to the one with beam on. In other words, the electron beam made no obvious difference for the sample size range we tested in this work. This is understandable, as the temperature rise in the sample is small for several reasons. First of all, the electron beam irradiating on the samples has a relatively low intensity. In addition, there is a large heat-conducting tungsten grip in intimate contact with the small sample. Also, the T g of the order of 700 K of this MG is significantly higher than room temperature. Moreover, the electron beam effect on the metallic bonds in the MG is not expected to be as significant as that on the directional and localized covalent bonds [33] . The possible contribution of beam-enhanced diffusion on surfaces is insignificant to alter the overall behaviour for the sample sizes used in this study. Therefore, for the beam-off samples, it is reasonable to convert the stress versus displacement curves to stress versus strain curves by assuming that their moduli remain identical to the sample with beam on ( Figure 3a ). It is worth noting that the displacement data plotted in Supplementary Figure S2 also contained the contributions from outside the gauge part and therefore should not be used directly to calculate the strain. Otherwise, the strain would be overestimated. How to cite this article: Tian, L. et al . Approaching the ideal elastic limit of metallic glasses. Nat. Commun. 3:609 doi: 10.1038/ncomms1619 (2012).